Exciton-dominated optical response of ultra-narrow graphene nanoribbons Narrow graphene nanoribbons exhibit substantial electronic bandgaps and optical properties fundamentally different from those of graphene. Unlike graphene—which shows a wavelength-independent absorbance for visible light—the electronic bandgap, and therefore the optical response, of graphene nanoribbons changes with ribbon width. Here we report on the optical properties of armchair graphene nanoribbons of width N =7 grown on metal surfaces. Reflectance difference spectroscopy in combination with ab initio calculations show that ultranarrow graphene nanoribbons have fully anisotropic optical properties dominated by excitonic effects that sensitively depend on the exact atomic structure. For N =7 armchair graphene nanoribbons, the optical response is dominated by absorption features at 2.1, 2.3 and 4.2 eV, in excellent agreement with ab initio calculations, which also reveal an absorbance of more than twice the one of graphene for linearly polarized light in the visible range of wavelengths. Graphene nanoribbons (GNRs) are raising great interest as they exhibit width-dependent sizable band gaps [1] suitable for digital electronics and optoelectronics [2] , while maintaining electron conjugation and the outstanding transport properties of graphene [3] . Furthermore, spin-polarized edge states for specific edge terminations [4] , [5] , [6] , tunable thermoelectric properties [7] as well as optical properties that are entirely dominated by the interacting photo-excited electron-hole pairs [8] , [9] , [10] , [11] are predicted. However, to maintain structural precision at the atomic level, including edge morphology, is clearly a challenge and requires structural control that goes far beyond the resolution of existing top–down approaches [2] . For some prototypical GNRs, this has recently been achieved using a bottom-up approach based on the covalent assembly of suitably designed molecular precursors [12] . The characterization of their electronic [13] , [14] and transport [15] properties revealed substantial band gaps that fully confirm the predictions [13] , [16] . This opens a way to tailor precise structural arrangements in the regime of ultranarrow GNRs and to realize specific edge terminations. Furthermore, recent studies showed that the bottom-up fabrication of GNRs can also be achieved in solution [17] , [18] where, although aggregation issues need to be addressed, the process can be easily scaled up. Similar as for their electronic properties, GNRs are expected to exhibit optical properties that are significantly different from the parent material graphene: Whereas graphene, owing to its linear band dispersion, reveals a wavelength-independent light absorbance of 2.3% [19] in the visible range, GNRs are expected to exhibit characteristic absorption bands related to band gap openings as well as to pronounced excitonic effects [8] , [9] , [10] , [11] that become dominant for quasi one-dimensional (1D) systems [20] . Here we characterize the optical properties of GNRs fabricated on metal substrates by means of reflectance difference spectroscopy (RDS) [21] and compare the results with ab-initio calculations including many-body effects. In this way we access the fundamental features of interacting photo-excited electron-hole pairs in an extreme regime of confinement and find an optical absorbance that is increased by a factor of ~2.4 as compared with graphene for visible linearly polarized light. Moreover, we catch the GNR in the act of its formation by following the signatures of fundamental optical excitations from the isolated molecular components through polymerization via intermolecular C–C coupling to the final GNR structure obtained after intramolecular cyclodehydrogenation. Optical spectroscopy of aligned GNRs We focus on the optical properties of armchair GNRs of width N =7 (7-AGNR, 0.74 nm wide with respect to edge C atoms, Fig. 1b ) as resulting from the bottom-up fabrication process on gold substrates [12] . RDS is a powerful technique sensitive to the optical anisotropy of a sample, that is, the reflectance difference Δ r for light polarized along two orthogonal directions x and y ( Fig. 1a ) (see Methods). It is thus perfectly suited to detect the anisotropic absorption of GNRs, provided that unidirectional alignment over macroscopic length scales can be achieved. This is obtained by depositing molecular precursors on the regularly stepped Au(788) surface, which results in a high degree of GNR alignment along the direction, with an average estimated nanoribbon length of 20 nm and a coverage around 0.8 monolayers (MLs) [13] , [22] , corresponding to an average distance between ribbon axes of ~1.4 nm. Both inter-ribbon interactions and finite-size effects are thus expected to be negligible (see Supplementary Note 1 ). In Fig. 1c (top and middle panels) we report the real and imaginary parts of the RD spectra for uniaxially aligned 7-AGNRs. To extract the differential dielectric response Δ ε of the ribbon, we apply the standard three-phase model (see Methods). The result is shown by the symbols in the bottom panel of Fig. 1c . We have further modelled the RD spectra and Δ ε by assuming a limited number of discrete optical transitions described by damped harmonic oscillators (see Methods). With only three such transitions, the experimental data can be fitted with remarkable accuracy (solid lines in Fig. 1c ; see also Supplementary Fig. 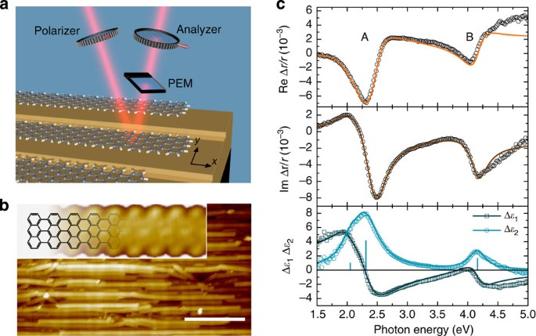Figure 1: RDS of aligned GNRs. (a) Schematic of the RDS experiment on uniaxially aligned 7-AGNRs on a vicinal surface. (b) STM topography image (Usample=−1.5 V; scale bar, 20 nm) of aligned 7-AGNRs grown on Au(788). The inset shows a small-scale STM image (Usample=−2.2 V; 4.1 × 1.2 nm2) and the chemical structure of a hydrogen-terminated 7-AGNR. (c) Measured (open circles) and fitted (solid lines) RD spectra of 7-AGNR on Au(788) measuredin situafter GNR synthesis. The RD spectrum of the pristine Au substrate has been subtracted. The bottom panel shows the differential dielectric function Δεobtained from the RD spectrum by applying the three-phase model (open symbols) and the fit to a model including three discrete harmonic oscillator transitions (lines). The blue bars indicate the energy position and oscillator strength (maximum ofε2≈Am/(EmΓm)) of the determined optical transitions (see Methods). 1 and Supplementary Table 1 ). This analysis allows us to interpret the anisotropy data in terms of optical excitations of the GNRs in the directions parallel and perpendicular to the GNR axis. We find that the differential dielectric response Δ ε 2 ( Fig. 1c , bottom panel) is dominated by three positive peaks at 2.1, 2.3 and 4.2 eV, respectively. The positive sign of Δ ε 2 indicates that these features can be ascribed to the absorption of light polarized along the ribbon axis. No relevant features are found, instead for light polarized in the perpendicular direction, as observed in other quasi-1D systems, including carbon nanotubes (CNTs) [23] . This confirms that we deal with highly unidirectional optical excitations. Figure 1: RDS of aligned GNRs. ( a ) Schematic of the RDS experiment on uniaxially aligned 7-AGNRs on a vicinal surface. ( b ) STM topography image ( U sample =−1.5 V; scale bar, 20 nm) of aligned 7-AGNRs grown on Au(788). The inset shows a small-scale STM image ( U sample =−2.2 V; 4.1 × 1.2 nm 2 ) and the chemical structure of a hydrogen-terminated 7-AGNR. ( c ) Measured (open circles) and fitted (solid lines) RD spectra of 7-AGNR on Au(788) measured in situ after GNR synthesis. The RD spectrum of the pristine Au substrate has been subtracted. The bottom panel shows the differential dielectric function Δ ε obtained from the RD spectrum by applying the three-phase model (open symbols) and the fit to a model including three discrete harmonic oscillator transitions (lines). The blue bars indicate the energy position and oscillator strength (maximum of ε 2 ≈ A m /( E m Γ m )) of the determined optical transitions (see Methods). Full size image Understanding excitonic effects To gain further insight into the nature of the low-energy peaks observed experimentally, we carried out state-of-the-art many-body perturbation theory [24] calculations for free-standing 7-AGNRs (see Methods). This allows us to take into account from first principles both electron–electron, within the GW approximation (refs 25 , 26 ) and electron–hole interactions, by solving the Bethe-Salpeter equation (BSE) (refs 27 , 28 ). Such effects are known to dominate electronic and optical excitations in such low-dimensional systems [20] . Image charge (IC) corrections [29] , [30] are included a posteriori to account for the polarization of the metallic substrate. Despite its simplicity, the IC approximation has proven successful to evaluate both the fundamental electronic [29] and optical [30] , [31] gaps in weakly coupled systems. The first-principles optical response ( ε 2 ) computed for the isolated 7-AGNR is shown in Fig. 2a . The spectrum is dominated by the response along the ribbon axis (solid curve), consistent with the strong anisotropy of the system, and shows three main features located at ~1.9, 2.3 and 4.1 eV, which are in excellent agreement with the experimental findings ( Fig.1c ). The computed data thus confirm two low-energy excitonic contributions at around 2.0 eV (the first one bearing most of the spectral weight, as shown by the vertical bars indicating the oscillator strength), which arise from optical transitions between the last valence and first conduction bands ( E 11 ), and the next to last valence and second conduction bands ( E 22 ), respectively (see Fig. 2a , right panel). Their exciton binding energies, defined as the difference between the energy of the optical excitation and the fundamental electronic gap, are 1.8 and 1.4 eV for the E 11 and E 22 excitations, respectively. These excitations correspond to Wannier-like quasi-1D excitons, fully delocalized along the ribbon width and with a spatial distribution along the ribbon axis entirely determined by the Coulomb interaction (see Fig. 2b ). These general features are also found in other π-conjugated 1D carbon systems, such as CNTs [32] , [33] , [34] and polymer chains [35] . Indeed, GNRs can be thought of as unrolled CNTs. Despite similar general features, the optical response of CNTs also shows significant differences. For instance, the spectra of CNTs with size comparable to that of the 7-AGNR are dominated by curvature-induced sp 2 –sp 3 rehybridization [32] . Moreover, low-lying dark-state excitations [34] , [36] are known to affect the CNT quantum yield [37] , while those dark states are not present in AGNRs in view of their different symmetry [9] . 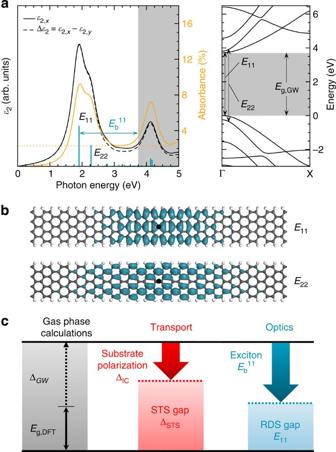Figure 2: Calculated optical response of 7-AGNRs. (a) Optical absorption spectrum and electronic band structure of 7-AGNRs calculated from first principles within theGW-BSE approach. The blue bars indicate the energy position and oscillator strength of the calculated optical excitations. The spectrum was obtained with a broadening of 0.5 eV and the same spectral lineshape used for fitting the RDS data (see Methods). The absolute absorbance for full coverage and light polarized along the longitudinal (x) direction is also shown (orange curve), as compared with the reference value of 2.3% for ML graphene (dotted orange line). (b) Exciton wavefunctions of the first and second excitons for 7-AGNRs. The calculated electron distribution is shown at fixed hole position (black dot). (c) Schematics of the relations between transport and optical gaps determined by STS and RDS, as compared withab-initiocalculations in vacuum. Figure 2: Calculated optical response of 7-AGNRs. ( a ) Optical absorption spectrum and electronic band structure of 7-AGNRs calculated from first principles within the GW -BSE approach. The blue bars indicate the energy position and oscillator strength of the calculated optical excitations. The spectrum was obtained with a broadening of 0.5 eV and the same spectral lineshape used for fitting the RDS data (see Methods). The absolute absorbance for full coverage and light polarized along the longitudinal ( x ) direction is also shown (orange curve), as compared with the reference value of 2.3% for ML graphene (dotted orange line). ( b ) Exciton wavefunctions of the first and second excitons for 7-AGNRs. The calculated electron distribution is shown at fixed hole position (black dot). ( c ) Schematics of the relations between transport and optical gaps determined by STS and RDS, as compared with ab-initio calculations in vacuum. Full size image The good agreement between theory and experiment concerning the energy positions confirms that the substrate has only a minor influence on the optical gap of 7-AGNRs, as expected in the case of weak hybridization [30] (see Supplementary Note 2 and 3 ). To compare with the remarkable optical absorption of a single graphene sheet (2.3 %), we also compute the absolute absorbance of an ML of 7-AGNRs (see Methods). In contrast to the wavelength-independent absorbance of graphene ( Fig. 2a , orange dotted line), here we find a strongly anisotropic absorbance ( Fig. 2a , orange curve), both in terms of wavelength and light polarization, because a significant spectral weight is transferred to the visible range by gap opening and excitonic effects. As a consequence, the absorbance of 7-AGNRs is increased by a factor of ~2.4 with respect to graphene when probing the system with visible light polarized along the ribbon axis. In view of technological applications, it is noteworthy that the range of frequencies with high absorbance can be tuned simply by changing the molecular precursor, and thus the width and the electronic and optical gaps of the material. Comparison of optical RD spectra with scanning tunnelling spectroscopy (STS) data recorded for 7-AGNRs with identical environment [13] reveals that both the optical and the transport gap (2.1 and 2.3 eV, respectively) have a similar magnitude ( Table 1 ). This a priori unexpected result can be understood from our theoretical calculations. Indeed, starting from the calculated electronic gap of the isolated ribbon (3.7 eV), the optical gap of the GNR on the substrate is obtained by including excitonic effects only, as substrate effects are expected to be negligible [30] . STS spectra must instead be corrected by including a significant IC contribution accounting for the substrate-induced polarization [13] ( Fig. 2c ). In fact, the calculated corrections turn out to be very similar ( Table 1 ), indicating that polarization effects are about as important as the exciton binding energy. A similar behaviour has previously been observed for CNTs adsorbed on Au(111) [38] . Table 1 Electronic and optical properties of 7-AGNRs and PA oligomers. Full size table On-surface reaction monitoring A powerful feature of RDS is that it permits to follow the bottom-up fabrication of GNRs in situ [39] . Indeed, we are able to monitor by RDS the full fabrication process step by step, from the deposition of the precursor molecules ( Fig. 3a , top) to on-surface polymerization ( Fig. 3a , middle) until the final formation of planar GNRs via cyclodehydrogenation ( Fig. 3a , bottom). 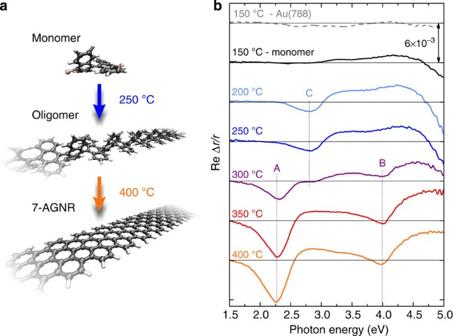Figure 3:In-situRDS monitoring of the bottom-up formation of GNRs. (a) Reaction scheme showing the evolution from the precursor monomer to atomically precise 7-AGNRs. (b) RD spectra recorded during 7-AGNR synthesis on Au(788). The black curve is obtained after deposition of ~0.8 ML of precursor monomers on Au(788). Coloured curves correspond to successively higher annealing temperatures to induce polymerization and finally cyclodehydrogenation into planar, straight 7-AGNRs. Figure 3b shows the evolution of the real part of the RD signal, as recorded during the preparation of 7-AGNRs. Focusing on the low-energy region, we note that the almost featureless spectrum of the precursor monomer evolves into a prominent peak C at 2.8 eV (light blue curve) on annealing, which corresponds to the formation of the polyanthrylene (PA). As the temperature increases, peak C disappears while new optical features develop, both at lower (2.3 eV, peak A ) and higher energies (4.0 eV, peak B ). Scanning tunnelling microscopy (STM) results confirm that this stage corresponds to the formation of the fully planar, aromatic 7-AGNRs (orange curve) via cyclodehydrogenation of the intermediate PA oligomers. The cyclodehydrogenation process, whose onset is found at 270 °C by real-time monitoring of the RD signal on annealing (see Supplementary Fig. 2 ), is fully completed at 400 °C. Figure 3: In-situ RDS monitoring of the bottom-up formation of GNRs. ( a ) Reaction scheme showing the evolution from the precursor monomer to atomically precise 7-AGNRs. ( b ) RD spectra recorded during 7-AGNR synthesis on Au(788). The black curve is obtained after deposition of ~0.8 ML of precursor monomers on Au(788). Coloured curves correspond to successively higher annealing temperatures to induce polymerization and finally cyclodehydrogenation into planar, straight 7-AGNRs. Full size image Optical and electronic properties of intermediate oligomers To characterize the individual steps of the reaction, we focus on the optical properties of the intermediate PA oligomers and compare them with the ones of the GNRs. 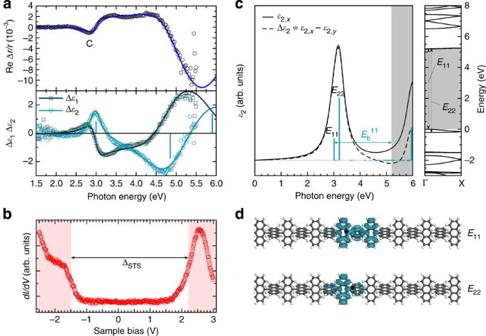Figure 4: Optical and tunnelling spectra of the PA oligomer. (a) Measured RD spectra (open circles) and three-phase model fit (solid lines) of PA oligomers formed by polymerization of the molecular precursors on Au(788) at 200 °C. The RD spectrum of the pristine Au substrate has been subtracted. The bottom panel shows the dielectric function of the simulated RD spectrum obtained by applying the three-phase model. The blue bars indicate the energy position and oscillator strength of the determined optical transitions. (b) Tunnelling spectrum recorded on the oligomer, revealing an electronic band gapΔSTSof 3.7 eV. (c) Optical absorption spectrum and electronic band structure of the oligomer calculated from first principles within theGW-BSE approach. The spectrum has been obtained using a broadening of 0.5 eV and the same spectral lineshape used for fitting the RDS data (see Methods). (d) Calculated exciton wavefunctions of the first and second excitons for the oligomer: the electron distribution is shown at fixed hole position (black dot). Figure 4a shows the real part of the RD spectrum for the PA oligomer, together with the differential dielectric response obtained with the three-phase model. Three peaks are needed to accurately fit the experimental data (see Supplementary Note 4, Supplementary Figure 3 , and Supplementary Table 2 ): two positive peaks at 3.0 and 5.9 eV, and a broad negative one at 4.8 eV, where the positive (negative) sign indicates that the features can be ascribed to the absorption of light polarized along (perpendicular to) the oligomer axis. The ab-initio GW -BSE absorption spectrum for the isolated PA oligomer is reported in Fig. 4c . For incident light polarized along the polymer axis ( x ), the computed optical onset is found at ~3.2 eV (again made of two individual excitations at 3.0 and 3.2 eV, see Fig. 4c ), while a second strong feature is located at ~6.0 eV. Instead, for light polarized along the transverse direction ( y ), a series of non-negligible excitations appears above 4.6 eV, but with intensities much lower than for the other polarization. Although the assignment of these features to the y -polarized experimental peak at 4.8 eV may be tentative, the agreement between theory and experiment for x -polarized light is striking. Note that both the fundamental electronic gap (5.3 eV) and the binding energy of the first exciton E 11 (2.3 eV) are found to be larger than those of the 7-AGNR (3.7 and 1.8 eV, respectively). This arises from the reduced π-conjugation of the oligomer compared with the ribbon, which is due to the non-planarity of adjacent anthracene units induced by steric repulsion, and the corresponding drastic reduction of the band dispersion. This can be clearly seen also from a comparison of exciton wavefunctions: the excitons of the oligomer are still Wannier-like ( Fig. 4d ), but extend over very few anthracene units (that is, ~1 nm), while they are significantly more delocalized for the ribbon ( Fig. 2b ), where π -conjugation is fully established. Figure 4: Optical and tunnelling spectra of the PA oligomer. ( a ) Measured RD spectra (open circles) and three-phase model fit (solid lines) of PA oligomers formed by polymerization of the molecular precursors on Au(788) at 200 °C. The RD spectrum of the pristine Au substrate has been subtracted. The bottom panel shows the dielectric function of the simulated RD spectrum obtained by applying the three-phase model. The blue bars indicate the energy position and oscillator strength of the determined optical transitions. ( b ) Tunnelling spectrum recorded on the oligomer, revealing an electronic band gap Δ STS of 3.7 eV. ( c ) Optical absorption spectrum and electronic band structure of the oligomer calculated from first principles within the GW -BSE approach. The spectrum has been obtained using a broadening of 0.5 eV and the same spectral lineshape used for fitting the RDS data (see Methods). ( d ) Calculated exciton wavefunctions of the first and second excitons for the oligomer: the electron distribution is shown at fixed hole position (black dot). Full size image Similar to that for the GNRs, we have also performed STS measurements on PA oligomers, which reveal an electronic band gap of 3.7 eV on the metal substrate (see Fig. 4b ). In this case the optical and electronic gaps differ by as much as 0.7 eV. On the theory side, the GW gap of 5.3 eV for the isolated oligomers is estimated to decrease on the substrate by 1.0–1.4 eV by the IC contribution (see Methods), in good agreement with experiments ( Table 1 ). The exciton binding energy of the lowest active exciton amounts to about 2.3 eV for the oligomer in vacuum. In general, substrate polarization and excitonic effects have a totally different nature. Consequently, the similarity of the optical and transport gaps found for the 7-AGNR on Au substrates is clearly fortuitous and specific to the confinement of neutral (excitons) and charged (quasi-particles) excitations of that system. In the oligomer case the cancellation of the two effects is not complete and results in a sensible difference between the two gaps (3.0 versus 3.7 eV for the experimental optical and transport gaps, respectively). RDS has been used to detect optical excitations of uniaxially oriented GNRs on gold, which are caught in the act of their formation. We find sensitive changes of the optical properties during the on-surface synthesis of 7-AGNRs. The optical spectra of both GNRs and the intermediate PA oligomers are found to be dominated by strongly anisotropic features in the visible range that are of excitonic nature, as elucidated by ab-initio calculations beyond density functional theory (DFT). Experimentally, the GNR optical gap turns out to be very similar to the transport gap as determined by STS. Far from indicating negligible excitonic effects, this results from an incidental compensation between substrate-induced polarization effects and large lowest exciton binding energy, which is not the case for the PA oligomers. Our results demonstrate that achieving the limit of atomically precise GNRs allows engineering of specific optical features in the visible range, and predict an enhancement of the optical absorbance by a factor of ~2.4 as compared with ML graphene for visible linearly polarized light. This opens the field for optical and optoelectronic applications that build on tailor-made optical properties of GNRs. Experimental procedures 7-AGNRs were grown on Au(788) as described in refs 12 , 13 . The metal substrate has been prepared by repeated sputtering with 1 keV Ar + ions and subsequent annealing at 740 K. Dibromo-bianthryl precursor monomers [12] were then deposited via ultrahigh vacuum sublimation from a heated quartz crucible on the pristine Au(788) substrate held at 423 K, and the sample was subsequently annealed at 673 K. This procedure yielded samples with a high coverage (~0.8 MLs, where a full ML corresponds to a densely packed GNR layer on Au(111)) of uniaxially aligned GNRs as shown in ref. 13 . STM was performed using a variable-temperature STM from Omicron Nanotechnology GmbH in constant current mode. GNR fabrication was also studied in situ by RDS. RD spectra were recorded of the pristine Au(788) sample, after monomer deposition, during annealing, and after cooling the sample. RDS is an optical method sensitive to the in-plane optical anisotropy of a sample [21] . RDS measures the normalized complex reflectance difference at normal incidence for light polarized along two orthogonal directions x and y ( Fig. 1b ). For optically isotropic crystals such as Au, the RD signal originates solely from the near-surface region; the bulk contribution to the RD signal is zero owing to the cubic symmetry of the fcc bulk crystal [21] . The RD spectrometer (ISA Jobin Yvon) used in this study (schematic see Fig. 1a ) allows recording the optical anisotropy in the energy range between 1.5 and 5.5 eV. A strain-free quartz viewport (Bombco Inc.) mounted on the ultrahigh vacuum preparation chamber allowed optical access to the sample at normal incidence. The x and y directions of the RD spectrometer (see Fig. 1a ) correspond to the and axes of the Au(788) sample, respectively. Modelling of RD spectra RD spectra of thin films on isotropic substrates are analysed using the so-called three-phase model [21] . According to this linear approximation of Δ r / r (given by the Fresnel equations), the RD signal of a thin film of thickness d and anisotropic dielectric function on top of an isotropic substrate with dielectric function is given by if the wavelength of the light λ ≫ d . Note that for absorbing substrates ( ε 2,b ≠0) such as Au, the real and imaginary part of the RD spectrum are affected by both Δ ε 1 and Δ ε 2 . However, as the real and imaginary part of Δ r / r are measured simultaneously, the above equation can be used to extract Δ ε from the RD spectrum if d and ε b are known. The anisotropic dielectric properties Δ ε of the GNRs were modelled using a sum of N damped harmonic oscillator transitions [40] yielding . The energetic position E m , width Γ m and amplitude A m of the transitions m =1… N were determined by fitting the model to the experimental data. Here A m >0 and A m <0 correspond to transitions polarized along the and directions, that is, along and perpendicular to the GNRs, respectively. For the calculation of the RD spectra, the GNR layer thickness was assumed to be 0.3 nm, while the dielectric function of the Au substrate was taken from au_2 of WVASE32 database by J.A. Wollam Co., Inc. In the present case, however, the anisotropic Au surface layer contributes to the overall RD signal as well. Therefore, the RD spectrum of the pristine substrate was subtracted from the experimental spectra for fitting of the oscillator transitions. This is valid as long as the interaction of the Au substrate with the GNRs and the oligomer phase is weak (see Supplementary Notes 2 and 3 ), and if the thickness of the adlayer and the anisotropic Au surface layer are both much smaller than λ . Under these conditions, interference effects can be neglected and the total RD signal is just the sum of the contribution of the Au surface and the adlayer. Computational details The ground-state calculations were performed for the isolated systems by using a DFT approach, as implemented in the Quantum ESPRESSO package [41] . A plane wave basis set was used (50 Ry cutoff) with norm-conserving pseudopotentials and local-density approximation exchange-correlation (xc) functional. To improve the band structure description obtained at the DFT level and simulate the optical spectra, electron–electron and electron–hole corrections are computed within the framework of many-body perturbation theory [24] . Quasi-particle corrections to the Kohn–Sham eigenvalues are calculated within the G 0 W 0 approximation for the self-energy operator, where the dynamic dielectric function was obtained within the plasmon-pole approximation. The Coulomb potential was hereafter truncated by using a box-shaped cutoff to remove the long-range interaction between periodic images and simulate isolated systems [42] . The optical absorption spectra were then computed as the imaginary part of the macroscopic dielectric function starting from the solution of the BSE. The static screening in the direct term was calculated within the random-phase approximation with inclusion of local field effects; the Tamm–Dancoff approximation for the BSE Hamiltonian was employed. The aforementioned many-body effects were included using the YAMBO code [43] , and further details can be found in refs 9 , 10 . For the evaluation of the optical absorbance, we assumed ML coverage, corresponding to a periodicity of 11 Å along the transverse direction. For the integration over the visible range, we considered the wavelength interval of 400–800 nm and checked the robustness of our result with respect to the smearing function. The effect of the substrate on the atomic structures and the ground-state electronic properties was checked for both the 7-AGNR and the oligomer. Band structures for the surface-supported systems are shown in Supplementary Fig. 4 and discussed in Supplementary Note 2 , demonstrating a weak interaction regime. The IC correction for the oligomer electronic gap has been computed following the procedure described in ref. 13 , and is further detailed in Supplementary Note 3 . How to cite this article: Denk, R. et al. Exciton-dominated optical response of ultra-narrow graphene nanoribbons. Nat. Commun. 5:4253 doi: 10.1038/ncomms5253 (2014).